Proposal for demonstrating the Hong–Ou–Mandel effect with matter waves The Hong–Ou–Mandel effect is a demonstration of destructive quantum interference between pairs of indistinguishable bosons, realised so far only with massless photons. Here we propose an experiment to realize this effect in the matter-wave regime using pair-correlated atoms produced via a collision of two Bose–Einstein condensates and subjected to two laser-induced Bragg pulses. We formulate a measurement protocol for the multimode matter-wave field, which—unlike the typical two-mode optical case—bypasses the need for repeated measurements under different displacement settings of the beam splitter, markedly reducing the number of experimental runs required to map out the interference visibility. Although the protocol can be used in related matter-wave schemes, we focus on condensate collisions. By simulating the entire experiment, we predict a Hong–Ou–Mandel dip visibility of ~69%. This visibility highlights strong quantum correlations between the atoms, paving the way for a possible demonstration of a Bell inequality violation with massive particles in a related Rarity–Tapster setup. Since its first demonstration, the Hong–Ou–Mandel (HOM) effect [1] has become a textbook example of quantum mechanical two-particle interference using pairs of indistinguishable photons. When two such photons enter a 50:50 beam splitter, with one photon in each input port, they both preferentially exit from the same output port, even though each photon individually had a 50:50 chance of exiting through either output port. The HOM effect was first demonstrated using optical parametric down-conversion [1] ; the same setup, but with an addition of linear polarisers, was subsequently used to demonstrate a violation of a Bell inequality [2] that is of fundamental importance to validating some of the foundational principles of quantum mechanics such as quantum nonlocality and long-distance entanglement. The HOM effect is a result of destructive quantum interference in a (bosonic) twin-photon state that leads to a characteristic dip in the photon coincidence counts at two photodetectors placed at the output ports of a beam splitter. The destructive interference occurs between two indistinguishable paths corresponding to the photons being both reflected from, or both transmitted through, the beam splitter. Apart from being of fundamental importance to quantum physics, the HOM effect underlies the basic entangling mechanism in linear optical quantum computing [3] , in which a twin-photon state |1,1› is converted into a quantum superposition —the simplest example of the elusive ‘NOON’ state [4] . Whereas the HOM effect with (massless) photons has been extensively studied in quantum optics (see refs 5 , 6 and references therein), two-particle quantum interference with massive particles remains largely unexplored. A matter-wave demonstration of the HOM effect would be a major advance in experimental quantum physics, enabling an expansion of foundational tests of quantum mechanics into previously unexplored regimes. Here we propose an experiment that can realize the HOM effect with matter waves using a collision of two atomic Bose–Einstein condensates (BECs) (as in refs 7 , 8 , 9 , 10 , 11 ) and a pair of laser-induced Bragg pulses. The HOM interferometer uses pair-correlated atoms from the scattering halo that is generated during the collision through the process of spontaneous four-wave mixing. The pair-correlated atoms are mixed using two separate Bragg pulses [12] , [13] that realize an atom-optics mirror and beam-splitter elements—in analogy with the use of twin-photons from parametric down-conversion in the optical HOM interferometer scheme. The HOM effect is quantified via the measurement of a set of atom–atom pair correlation functions between the output ports of the interferometer. Using stochastic quantum simulations of the collisional dynamics and the application of Bragg pulses, we predict a HOM dip visibility of ~69% for realistic experimental parameters. A visibility larger than 50% is indicative of stronger than classical correlations between the atoms in the scattering halo [7] , [11] , [14] , [15] , [16] , which in turn renders our system as a suitable platform for demonstrating a Bell's inequality violation with matter waves using a closely related Rarity–Tapster scheme [17] . Setup The schematic diagram of the proposed experiment is shown in Fig. 1 . A highly elongated (along the x axis) BEC is initially split into two equal and counterpropagating halves travelling with momenta ± k 0 along z in the centre-of-mass frame. Constituent atoms undergo binary elastic collisions that produce a nearly spherical s -wave scattering halo of radius (ref. 8 ) in momentum space due to energy and momentum conservation. The elongated condensates have a disk-shaped density distribution in momentum space, shown in Fig. 1b on the north and south poles of the halo. After the end of the collision (which in this geometry corresponds to complete spatial separation of the condensates in position space), we apply two counterpropagating lasers along the x axis whose intensity and frequency are tuned to act as a resonant Bragg π-pulse with respect to two diametrically opposing momentum modes, k 1 and k 2 =− k 1 , situated on the equatorial plane of the halo and satisfying | k 1,2 |= k r . 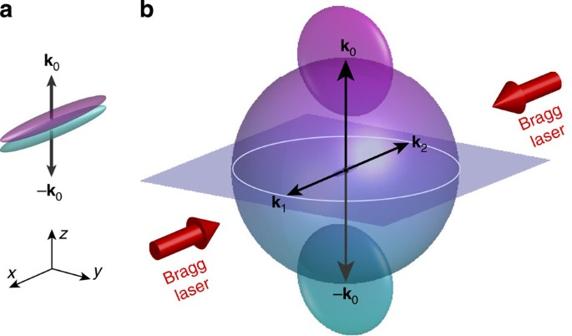Figure 1: Schematic diagram of the collision geometry. (a) Position space picture of two elongated (along thexaxis) BECs counterpropagating alongzwith equal but opposite momenta ±k0. (b) Momentum-space distribution of the atomic cloud showing the (disk shaped) condensates on the north and south poles of the spherical halo of scattered atoms (see text for further details). Figure 1: Schematic diagram of the collision geometry. ( a ) Position space picture of two elongated (along the x axis) BECs counterpropagating along z with equal but opposite momenta ± k 0 . ( b ) Momentum-space distribution of the atomic cloud showing the (disk shaped) condensates on the north and south poles of the spherical halo of scattered atoms (see text for further details). Full size image Previous experiments and theoretical work [7] , [9] , [10] , [11] , [18] , [19] , [20] , [21] , [22] , [23] have shown the existence of strong atom–atom correlation between such diametrically opposite modes, similar to the correlation between twin-photons in parametric down-conversion. Applying the Bragg π-pulse to the collisional halo replicates an optical mirror and reverses the trajectories of the scattered atoms with momenta k 1 and k 2 , and a finite region around them. We assume that the pulse is tuned to operate in the so-called Bragg regime of the Kapitza-Dirac effect [13] , [24] (diffraction of a matter wave from a standing light field), corresponding to conditions in which second- and higher-order diffractions are suppressed. The system is then allowed to propagate freely for a duration so that the targeted atomic wave-packets regain spatial overlap in position space. We then apply a second Bragg pulse—a π/2-pulse—to replicate an optical 50:50 beam splitter, which is again targeted to couple k 1 and k 2 , thus realising the HOM interferometer. The timeline of the proposed experiment is illustrated in Fig. 2a , whereas the results of numerical simulations (see Methods) of the collision dynamics and the application of Bragg pulses are shown in Fig. 2b–d : panel b shows the equatorial slice of the momentum-space density distribution n ( k , t ) of the scattering halo at the end of collision; panels c and d show the halo density after the application of the π and π/2 pulses, respectively. The ‘banana’ shaped regions in panel c correspond to ‘kicked’ populations between the targeted momenta around k 1 and k 2 in the original scattering halo, whereas panel d shows the density distribution after mixing. The density modulation in panel c is simply the result of interference between the residual and transferred atomic populations after the π-pulse upon their recombination on the beam splitter. The residual population is due to the fact that the pairs of off-resonance modes in these parts of the halo (which are coupled by the same Bragg pulses as they share the same momentum difference 2 k r as the resonant modes k 1 and k 2 ) no longer satisfy the perfect Bragg-resonance condition and therefore the population transfer during the π-pulse is not 100% efficient. As these components have unequal absolute momenta, their amplitudes accumulate a nonzero relative phase due to phase dispersion during the free propagation. The accrued relative phase results in interference fringes upon the recombination on the beam splitter, with an approximate period of . 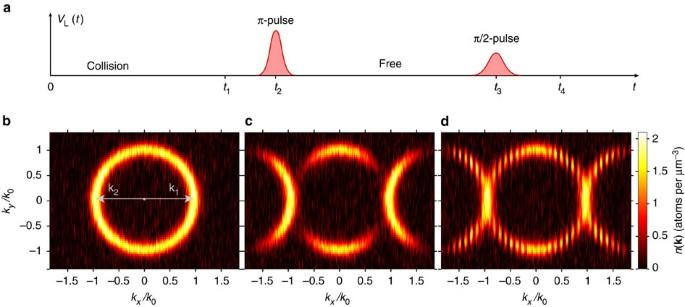Figure 2: Timeline of the proposed experiment and snapshots of the collisional halo from the numerical simulations. In panela, timet=0 corresponds to the coherent splitting of the source condensate that sets up the collision;VL(t) denotes the depth of the lattice potential formed by the Bragg lasers, with the first hump indicating the mirror (π) pulse, whereas the second hump indicates the beam-splitter (π/2) pulse (the initial source-splitting pulse is not shown for clarity). Panelsb–dshow the results of numerical simulations of the momentum-space density distributionn(k) of scattered atoms on the equatorial plane of the halo; panelbshows the density distribution after the collision, att1=65 μs; (c) shows the density distribution after the π-pulse, centred att2=75 μs and having a duration ofτπ=2.5 μs (r.m.s. width of Gaussian envelope); and (d) shows the density distribution after the final π/2-pulse, with Δtfree=t3−t2=85 μs and τπ/2=2.5 μs (see Methods for further details; the durations shown on the time axis are not to scale). The momentum axeskx,yin panelsb–dare normalized to the collision momentumk0≡|k0| (in wave-number units), which in our simulations wask0=4.7 × 106m−1. The simulations were carried out for an initial BEC containing a total ofN=4.7 × 104atoms of metastable helium (4He*), prepared in a harmonic trap of frequencies (ωx,ωy,ωz)/2π=(64, 1150, 1150) Hz, and colliding with the scattering length ofa=5.3 nm; all these parameters are very close to those realised in recent experiments7,8. Figure 2: Timeline of the proposed experiment and snapshots of the collisional halo from the numerical simulations. In panel a , time t =0 corresponds to the coherent splitting of the source condensate that sets up the collision; V L ( t ) denotes the depth of the lattice potential formed by the Bragg lasers, with the first hump indicating the mirror (π) pulse, whereas the second hump indicates the beam-splitter (π/2) pulse (the initial source-splitting pulse is not shown for clarity). Panels b – d show the results of numerical simulations of the momentum-space density distribution n ( k ) of scattered atoms on the equatorial plane of the halo; panel b shows the density distribution after the collision, at t 1 =65 μs; ( c ) shows the density distribution after the π-pulse, centred at t 2 =75 μs and having a duration of τ π =2.5 μs (r.m.s. width of Gaussian envelope); and ( d ) shows the density distribution after the final π/2-pulse, with Δ t free = t 3 − t 2 =85 μs and τ π/2 =2.5 μs (see Methods for further details; the durations shown on the time axis are not to scale). The momentum axes k x , y in panels b – d are normalized to the collision momentum k 0 ≡| k 0 | (in wave-number units), which in our simulations was k 0 =4.7 × 10 6 m −1 . The simulations were carried out for an initial BEC containing a total of N =4.7 × 10 4 atoms of metastable helium ( 4 He*), prepared in a harmonic trap of frequencies ( ω x , ω y , ω z )/2π=(64, 1150, 1150) Hz, and colliding with the scattering length of a =5.3 nm; all these parameters are very close to those realised in recent experiments [7] , [8] . Full size image Owing to the indistinguishability of the paths of the Bragg-resonant modes k 1 and k 2 through the beam splitter and the resulting destructive quantum interference, a measurement of coincidence counts between the atomic populations in these modes will reveal a suppression compared with the background level. To reveal the full structure of the HOM dip, including the background level where no quantum interference occurs, we must introduce path distinguishability between the k 1 and k 2 modes. One way to achieve this, which would be in a direct analogy with shifting the beam splitter in the optical HOM scheme, is to change the Bragg-pulse resonance condition from the ( k 1 , k 2 ) pair to ( k 1 , k 2 + ê x δk ), where ê x is the unit vector in the x -direction. The approach to the background coincidence rate between the populations in the k 1 and k 2 modes would then correspond to performing the same experiment for increasingly large displacements δk . Taking into account that acquiring statistically significant results for each δk requires repeated runs of the experiment (typically thousands), this measurement protocol could potentially pose a significant practical challenge because of the very large total number of experimental runs required. Proposed measurement protocol To overcome this challenge, we propose an alternative measurement protocol that can reveal the full structure of the HOM dip from just one Bragg-resonance condition, requiring only one set of experimental runs. The protocol takes advantage of the broadband, multimode nature of the scattering halo and the fact that the original Bragg-pulse couples not only the targeted momentum modes k 1 and k 2 , but also many other pairs of modes that follow distinguishable paths through the beam splitter. One such pair, k 3 =( k x , k y , k z )= k r (cos( θ ),sin( θ ),0) and k 4 =− k 3 , located on the halo peak, is shown in Fig. 3a and corresponds to a rotation by angle θ away from k 1 and k 2 . The modes k 3 and k 4 are equivalent to the original pair in the sense of their quantum statistical properties and therefore, these modes can be used for the measurement of the background level of coincidence counts, instead of physically altering the paths of the k 1 and k 2 modes. The angle θ now serves the role of the ‘displacement’ parameter that scans through the shape of the HOM dip. A topologically equivalent optical scheme is shown in Fig. 3b,c , which is in turn similar to the one analysed in the study by Rarity and Tapster [25] using a broadband source of angle-separated pair-photons and directionally asymmetric apertures. 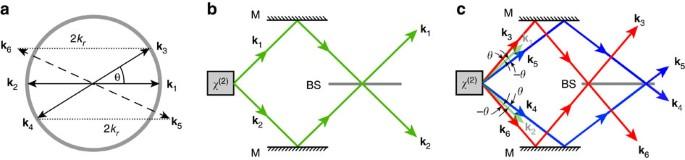Figure 3: Schematic of matter-wave momentum modes affected by the Bragg pulses and the topologically equivalent optical setups. In panela, the diametrically opposite vectorsk1andk2= −k1show the targeted momentum modes on the scattering halo; their amplitude is given by the halo peak radius,kr=|k1|=|k2|, which is equal tokr≃0.95|k0| in this part of the halo8. Also shown are the to-be-measured momentum componentsk3andk4corresponding to a rotation byθaway from the targeted modes, which couple, respectively, tok6=k3−2k1andk5=k4+2k1by the same Bragg pulses. Panelsbandcshow equivalent optical schemes that use aχ(2)nonlinear crystal that is optically pumped to produce twin-photons via parametric down-conversion. Inb, we depict the archetypal optical HOM setup that corresponds to the case ofθ=0 in the matter-wave scheme. A twin-photon state in modesk1andk2is first selected from a broadband source, then mixed at the beam splitter (BS) after reflection from the mirror (M), and photon coincidence counts are measured between the two symmetric output ports of the interferometer. Inc, we depict the optical setup that is equivalent toθ>0 in the mater-wave proposal. Two twin-photon states in (k3,k4) and in (k5,k6) are selected from the broadband source; the asymmetry of the pairs about the optical axis of the interferometer means that the correlated photons from the respective pairs will arrive at the beam splitter at spatially separate locations and will mix with photons from the other pair, which introduces distinguishability between the paths through the interferometer. Figure 3: Schematic of matter-wave momentum modes affected by the Bragg pulses and the topologically equivalent optical setups. In panel a , the diametrically opposite vectors k 1 and k 2 = − k 1 show the targeted momentum modes on the scattering halo; their amplitude is given by the halo peak radius, k r =| k 1 |=| k 2 |, which is equal to k r ≃ 0.95| k 0 | in this part of the halo [8] . Also shown are the to-be-measured momentum components k 3 and k 4 corresponding to a rotation by θ away from the targeted modes, which couple, respectively, to k 6 = k 3 −2 k 1 and k 5 = k 4 +2 k 1 by the same Bragg pulses. Panels b and c show equivalent optical schemes that use a χ (2) nonlinear crystal that is optically pumped to produce twin-photons via parametric down-conversion. In b , we depict the archetypal optical HOM setup that corresponds to the case of θ =0 in the matter-wave scheme. A twin-photon state in modes k 1 and k 2 is first selected from a broadband source, then mixed at the beam splitter (BS) after reflection from the mirror (M), and photon coincidence counts are measured between the two symmetric output ports of the interferometer. In c , we depict the optical setup that is equivalent to θ >0 in the mater-wave proposal. Two twin-photon states in ( k 3 , k 4 ) and in ( k 5 , k 6 ) are selected from the broadband source; the asymmetry of the pairs about the optical axis of the interferometer means that the correlated photons from the respective pairs will arrive at the beam splitter at spatially separate locations and will mix with photons from the other pair, which introduces distinguishability between the paths through the interferometer. Full size image In the proposed protocol, detection (after the final Bragg pulse) of atom coincidences at the pair of originally correlated momenta k 3 and k 4 corresponds to both paths being separately reflected on the beam splitter ( Fig. 3c ). Apart from this outcome, we need to take into account the coincidences between the respective Bragg-partner momenta, k 6 and k 5 (separated, respectively, from k 3 and k 4 by the same difference 2 k r as k 1 from k 2 ). Coincidences at k 6 and k 5 correspond to atoms of the originally correlated momenta k 3 and k 4 being both transmitted through the beam splitter ( Fig. 3c ). Finally, in order to take into account all possible channels contributing to coincidence counts between the two arms of the interferometer, we need to measure coincidences between k 3 and k 6 , as well as between k 4 and k 5 . This ensures that the total detected flux at the output ports of the beam splitter matches the total input flux. In addition to this, we normalize the bare coincidence counts to the product of single-detector count rates, that is, the product of the average number of atoms in the two output arms of the interferometer. We use the normalized correlation function as the total population in the four relevant modes varies as the angle θ is increased, implying that the raw coincidence rates are not a suitable quantity to compare at different angles. HOM effect and visibility of the dip With this measurement protocol in mind, we quantify the HOM effect using the normalized second-order correlation function after the π/2-pulse concludes at t = t 4 . Here, and correspond to the number of atoms detected, respectively, on the two (right and left) output ports of the beam splitter, with the detection bins centred around the four momenta of interest k i ( i =3, 4, 5 and 6), for any given angle θ ( Fig. 2e ). More specifically, is the atom number operator in the integration volume centred around k i , where is the momentum-space density operator, with and the corresponding creation and annihilation operators (the Fourier components of the field operators and , see Methods). The double-colon notation in indicates normal ordering of the creation and annihilation operators. The integrated form of the second-order correlation function, which quantifies the correlations in terms of atom number coincidences in detection bins of certain size rather than in terms of local density-density correlations, accounts for limitations in the experimental detector resolution, in addition to improving the signal-to-noise ratio that is typically low owing to the relatively low density of the scattering halo; in typical condensate collision experiments and in our simulations, the low density translates to a typical halo-mode occupation of ~0.1. We choose to be a rectangular box with dimensions corresponding to the r.m.s. width of the initial momentum distribution of the trapped condensate, which is a reasonable approximation to the mode (or coherence) volume in the scattering halo [10] , [22] . The second-order correlation function , quantifying the HOM effect as a function of the path-distinguishability angle θ , is shown in Fig. 4 . For θ =0, where k 3(4) = k 1(2) , we observe maximum suppression of coincidence counts relative to the background level because of the indistinguishability of the paths. As we increase | θ |>0, we no longer mix k 3 and k 4 as a pair and their paths through the beam splitter become distinguishable; the path interference is lost, and we observe an increase in the magnitude of the correlation function to the background level. We quantify the visibility of the HOM dip via , where occurs for θ =0 and for sufficiently large θ such that momenta k 5,6 lie outside the scattering halo. Owing to the oscillatory nature of the wings (see below) we take to correspond to the mean of for . Using this definition, we measure a visibility of , where the uncertainty of ±0.08 corresponds to taking into account the full fluctuations of about the mean in the wings rather than fitting the oscillations ( Supplementary Fig. 1 and Supplementary Notes 1 and 2 ). The visibility >0.5 is consistent with the nonclassical effect of violation of Cauchy–Schwarz inequality with matter waves [22] , observed recently in condensate collision experiments [11] . The exact relationship between the visibility and the Cauchy–Schwarz inequality is discussed further in Supplementary Note 3 , as are simple (approximate) analytic estimates of the magnitude of the HOM dip visibility ( Supplementary Notes 1–5 and Supplementary Fig. 2 ). 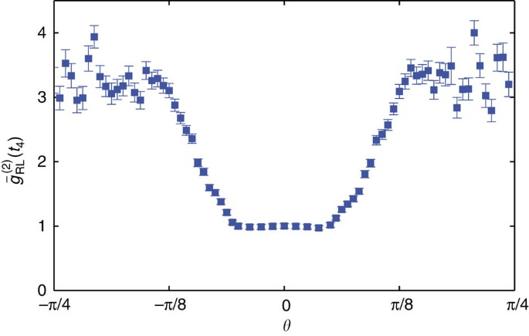Figure 4: HOM dip. Normalized atom–atom correlation functionbetween the two arms of the interferometer, characterizing the HOM effect as a function of the path-distinguishability angleθ. Error bars denote sampling error from ~30,000 stochastic simulations (see Methods). The atom counting bins are rectangular boxes with sidesδkx=0.01k0andδky,z=0.19k0, which approximate the widths of the momentum distribution of the initial trapped BEC. Figure 4: HOM dip. Normalized atom–atom correlation function between the two arms of the interferometer, characterizing the HOM effect as a function of the path-distinguishability angle θ . Error bars denote sampling error from ~30,000 stochastic simulations (see Methods). The atom counting bins are rectangular boxes with sides δk x =0.01 k 0 and δk y , z =0.19 k 0 , which approximate the widths of the momentum distribution of the initial trapped BEC. Full size image Width of the HOM dip The broadband, multimode nature of the scattering halo implies that the range of the path-length difference over which the HOM effect can be observed is determined by the spectral width of the density profile of the scattering halo. Therefore, the width of the HOM dip is related to the width of the halo density. This is similar to the situation analysed in Rarity and Tapster [25] using pair-photons from a broadband parametric down-converter. The angular width of the HOM dip extracted from Fig. 4 is approximately radians, which is indeed close to the width (full width at half maximum) of the scattering halo in the relevant direction, radians (see also Supplementary Note 2 for simple analytic estimates). The same multimode nature of the scattering halo contributes to the oscillatory behaviour in the wings of the HOM dip profile: here we mix halo modes with unequal absolute momenta and the resulting phase dispersion from free propagation leads to oscillations similar to those observed with two-colour photons [25] . Comparison with optical parametric down-conversion We emphasize that the input state in our matter-wave HOM interferometer is subtly different from the idealized twin-Fock state |1,1› used in the simplest analytic descriptions of the optical HOM effect. This idealized state stems from treating the process of spontaneous optical parametric down-conversion (SPDC) in the weak-gain regime. We illustrate this approximation by considering a two-mode toy model of the process, which in the undepleted pump approximation is described by the Hamiltonian that produces perfectly correlated photons in the â 1 and â 2 modes, where is a gain coefficient related to the quadratic nonlinearity of the medium and the amplitude of the coherent pump beam. (In the context of condensate collisions, the coupling corresponds to at the same level of ‘undepleted pump’ approximation [10] , [22] ; see Methods for the definitions of U and ρ 0 .) The full output state of the SPDC process in the Schrödinger picture is given by , where α =tanh( gt ) and t is the interaction time [26] . In the weak-gain regime, corresponding to , this state is well approximated by , that is, by truncating the expansion of and neglecting the contribution of the |2,2› and higher n components. This regime corresponds to mode populations being much >1, . The truncated state itself is qualitatively identical to the idealized state |1,1› as an input to the HOM interferometer: both result in a HOM dip minimum of and in the wings (where for the |1,1› case), with the resulting maximum visibility of V =1. If, on the other hand, the contribution of the |2,2› and higher n components is not negligible (which is the case, for example, of then the raw coincidence counts at the HOM dip and the respective normalized correlation function no longer equal to zero; in fact, the full SPDC state for arbitrary α <1 leads to a HOM dip minimum of and in the wings, which in turn results in a reduced visibility of . Despite this reduction, the visibility is still very close to V =1 in the weak-gain regime ( ), where it scales as . The process of four-wave mixing of matter waves gives rise to an output state analogous to the above SPDC state for each pair of correlated modes (see, for example, refs 10 , 22 and Supplementary Note 1 ). Indeed, the fraction of atoms converted from the source BEC to all scattering modes is typically <5%, which justifies the use of the undepleted pump approximation. The typical occupation numbers of the scattered modes are, however, beyond the extreme of a very weak gain. In our simulations, the mode occupation on the scattering halo is on the order of 0.1 and therefore, even in the simplified analytical treatment of the process, the output state of any given pair of correlated modes cannot be approximated by the truncated state |0,0›+ α |1,1› or indeed the idealized twin-Fock state |1,1›. Scaling with mode population and experimental considerations At the basic level, our proposal only relies on the existence of the aforementioned pair-correlations between scattered atoms, with the strength of the correlations affecting the visibility of the HOM dip. For a sufficiently homogeneous source BEC [22] , [27] , the correlations and thus the visibility V effectively depend only on the average mode population in the scattering halo, with a scaling of V on given by by our analytic model. Dependence of on system parameters such as the total number of atoms in the initial BEC, trap frequencies and collision duration is well understood both theoretically and experimentally [7] , [8] , [10] , [11] , and each can be sufficiently controlled such that a suitable mode population of can, in principle, be targeted. There lies, however, a need for optimization: very small populations are preferred for higher visibility, but they inevitably lead to a low signal to noise, hence requiring a potentially very large number of experimental runs for acquiring statistically significant data. Large occupations, on the other hand, lead to higher signal to noise, but also to a degradation of the visibility towards the nonclassical threshold of V =0.5. The mode population of ~0.1 resulting from our numerical simulations appears to be a reasonable compromise; following the scaling of the visibility with predicted by the simple analytic model, it appears that one could safely increase the population to ~0.2 before a nonclassical threshold is reached to within a typical uncertainty of ~12% (as per quoted value of ) obtained through our simulations. The proposal is also robust to other experimental considerations such as the implementation of the Bragg pulses; for example, one may use square Bragg pulses rather than Gaussians. Furthermore, experimental control of the Bragg pulses is sufficiently accurate to avoid any degradation of the dip visibility. Modifying the relative timing of the π and π/2 pulses by few percent in our simulations does not explicitly affect the dip visibility, rather only the period of the oscillations in the wings of . This may lead to a systematic change in the calculated dip visibility, however, this is overwhelmed by the uncertainty of 12% that accounts for the fluctuations of about the mean. Importantly, we expect that the fundamentally new aspects of the matter-wave setup, namely the multimode nature of the scattering halo and the differences from the archetypical HOM input state of |1,1›, as well as the specific measurement protocol we have proposed for dealing with these new aspects, are broadly applicable to other related matter-wave setups that generate pair-correlated atoms. These include molecular dissociation [19] , an elongated BEC in a parametrically shaken trap [14] , or degenerate four-wave mixing in an optical lattice [28] , [29] . In the present work, we focus on condensate collisions only because of the accurate characterization, both experimental and theoretical, of the atom–atom correlations, including in a variety of collision geometries [7] , [8] , [9] , [10] , [11] . In summary, we have shown that an atom-optics analogue of the HOM effect can be realised using colliding condensates and laser-induced Bragg pulses. The HOM dip visibility >50% implies that the atom–atom correlations in this process cannot be described by classical stochastic random variables. Generation and detection of such quantum correlations in matter waves can serve as precursors to stronger tests of quantum mechanics such as those implied by a Bell inequality violation and the Einstein–Podolsky–Rosen paradox [30] . In particular, the experimental demonstration of the atom-optics HOM effect would serve as a suitable starting point to experimentally demonstrate a violation of a Bell inequality using an atom-optics adaptation of the Rarity–Tapster setup [17] . In this setup, one would tune the Bragg pulses as to realize two separate HOM interferometer arms, enabling to mix two angle-resolved pairs of momentum modes from the collisional halo, such as ( k , q ) and (− k ,− q ), which would then form the basis of a Bell state (ref. 31 ). Stochastic Bogoliubov approach for simulations To simulate the collision dynamics, we use the time-dependent stochastic Bogoliubov approach [8] , [23] used previously to accurately model a number of condensate collision experiments [8] , [7] , [11] . In this approach, the atomic field operator is split into , where is the mean-field component describing the source condensates and is the fluctuating component (treated to lowest order in perturbation theory) describing the scattered atoms. The mean-field component evolves according to the standard time-dependent Gross–Pitaevskii equation, where the initial state is taken in the form of . This models an instantaneous splitting at t =0 of a zero-temperature condensate in a coherent state into two halves that subsequently evolve in free space, where ρ 0 ( r ) is the particle number density of the initial (trapped) sample before splitting. The fluctuating component is simulated using the stochastic counterpart of the Heisenberg operator equations of motion [8] , [22] , , in the positive P -representation with the vacuum initial state. Here represents the kinetic energy term, an effective mean-field potential, plus the lattice potential V BP ( r , t ) imposed by the Bragg pulses, whereas is an effective coupling responsible for the spontaneous pair-production of scattered atoms. The interaction constant U is given by U =4π ℏ 2 a / m , where m is the atomic mass and a is the s -wave scattering length. Details of Bragg pulses The Bragg pulses are realised by two interfering laser beams (assumed for simplicity to have a uniform intensity across the atomic cloud and zero relative phase) that create a periodic lattice potential , where V L ( t ) is the lattice depth and is the lattice vector determined by the wave vectors k L , i ( i =1, 2) of the two lasers, and tuned to | k L |= k r . The Bragg pulses couple momentum modes k i and k j = k i −2 k L , satisfying momentum and energy conservation (up to a finite width owing to energy-time uncertainty [24] ). The lattice depth is ramped up (down) according to , where t 2(3) is the pulse centre, whereas τ π(π/2) is the pulse duration that governs the transfer of atomic population between the targeted momentum modes: a π-pulse is defined by and converts the entire population from one momentum mode to the other, whereas a π/2-pulse is defined by and converts only half of the population. Aspects of measurement after expansion In practice, the atom–atom correlations quantifying the HOM interference are measured in position space after the low-density scattering halo expands ballistically in free space and falls under gravity onto an atom detector. The detector records the arrival times and positions of individual atoms, which is literally the case for metastable helium atoms considered here [7] , [8] , [9] , [11] , [32] . The arrival times and positions are used to reconstruct the three-dimensional velocity (momentum) distribution before expansion, as well as the atom–atom coincidences for any desired pair of momentum vectors. In our simulations and the proposed geometry of the experiment, the entire system (including the Bragg pulses) maintains reflectional symmetry about the yz -plane, with z being the vertical direction. Therefore, the effect of gravity can be completely ignored as it does not introduce any asymmetry to the momentum distribution of the atoms and their correlations on the equatorial plane of the halo or indeed any other plane parallel to it. How to cite this article: Lewis-Swan, R. J. & Kheruntsyan, K. V. Proposal for demonstrating the Hong–Ou–Mandel effect with matter waves. Nat. Commun. 5:3752 doi: 10.1038/ncomms4752 (2014).